Steroid hormone signalling links reproduction to lifespan in dietary-restrictedCaenorhabditis elegans Dietary restriction (DR) increases healthspan and longevity in many species, including primates, but it is often accompanied by impaired reproductive function. Whether signals associated with the reproductive system contribute to or are required for DR effects on lifespan has not been established. Here we show that expression of the cytochrome P450 DAF-9/CYP450 and production of the steroid hormone Δ 7 -dafachronic acid (DA) are increased in C. elegans subjected to DR. DA signalling through the non-canonical nuclear hormone receptor NHR-8/NHR and the nutrient-responsive kinase let-363 /mTOR is essential for DR-mediated longevity. Steroid signalling also affects germline plasticity in response to nutrient deprivation and this is required to achieve lifespan extension. These data demonstrate that steroid signalling links germline physiology to lifespan when nutrients are limited, and establish a central role for let-363 /mTOR in integrating signals derived from nutrients and steroid hormones. Dietary restriction (DR), defined as a reduction in nutrient intake without causing malnutrition, extends longevity in many species and generally improves health during advanced age [1] . In response to nutrient deprivation, animals may curtail energetically expensive processes such as reproduction. Although longevity and fertility can be uncoupled by altering the composition of the diet [2] , DR is usually associated with reduced and delayed fertility [3] . However, molecular networks that link longevity to fertility remain uncharacterized. These observations prompted us to investigate the effect of DR on the activity of a major ‘reproductive pathway’ in C. elegans : the steroid-signalling pathway. Here, we show that DR leads to increased production of dafachronic acids (DAs) and that this increase is required for lifespan extension. In response to nutrient scarcity, steroid signalling is mediated by the nuclear hormone receptor NHR-8 and links TOR signalling and germline plasticity to longevity. Taken together, our data suggest that diet-induced lifespan extension is part of a coordinated response that involves reproductive phenotypes. DR increases DA levels We first measured the effect of DR on expression of the cytochrome P450 enzyme DAF-9 and its products, the steroid hormones 7- and 4-cholesten-3-one-26-oic acids, also called Δ 7 - and Δ 4 -DAs. We found that transcription of daf-9 and production of Δ 7 -DA were both increased about six-fold on bacterial deprivation of wild-type animals ( Fig. 1a,b and Supplementary Fig. 1 ). A previous report has shown that DAs are produced in an insulin and TGFβ signalling-dependent manner in developing C. elegans under nutrient-favourable conditions [4] . However, we found that DR also induces daf-9 expression in adult mutants lacking functional insulin signalling ( daf-16 /FOXO mutant) or TGFβ signalling ( daf-5 /SKI and daf-7 /TGFβ; Supplementary Fig. 2 ). Thus, our observation that DAs are produced in gravid adult worms in response to starvation contrasts with the findings in developing worms. Interestingly, DAs are also produced upon ablation of the germline, an intervention that extends lifespan in both worms and flies [4] , [5] , [6] . 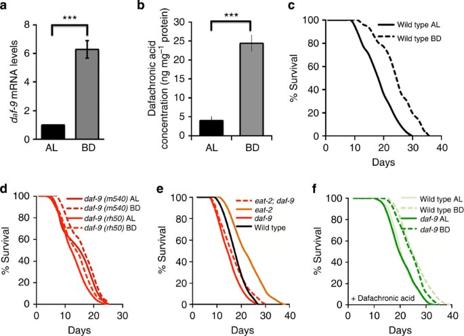Figure 1: DA production by DAF-9 is required for dietary restriction-mediated lifespan extension. (a,b)daf-9mRNA levels (a) and Δ7-DA levels (b) are increased on bacterial deprivation (BD) of wild-typeC. eleganscompared with animals fedad libitum(AL; ***P<0.001).n=3 independent biological samples for Δ7-DA measurements andn=9 independent biological samples fordaf-9mRNA quantification (ΔΔCt=−2.651575 normalized to AL). (c,d) Nutrient deprivation extends the mean lifespan of wild-type animals by 41% (c);P<0.0001) but does not affect the mean lifespan of animals carrying them540orrh50alleles ofdaf-9(d);P=0.02 andP=0.126, respectively). (e)eat-2(ad1116);daf-9(rh50)double mutants anddaf-9(rh50)single mutants exhibit similar mean lifespans (P=0.05). (f) Addition of 100 nM Δ7-DA does not affect the lifespan of wild-type animals under AL or BD conditions but restores the lifespan extension ofdaf-9(rh50)mutants (P<0.0001).Pvalues for survival analysis were calculated using the log-rank (Mantel–Cox) test.Pvalues for QRT–PCR data were calculated using the two-tailed Student’st-test; Error bars represent s.d. Lifespan values indicate mean±95% CI. Figure 1: DA production by DAF-9 is required for dietary restriction-mediated lifespan extension. ( a , b ) daf-9 mRNA levels ( a ) and Δ 7 -DA levels ( b ) are increased on bacterial deprivation (BD) of wild-type C. elegans compared with animals fed ad libitum (AL; *** P <0.001). n =3 independent biological samples for Δ 7 -DA measurements and n =9 independent biological samples for daf-9 mRNA quantification (ΔΔCt=−2.651575 normalized to AL). ( c , d ) Nutrient deprivation extends the mean lifespan of wild-type animals by 41% ( c ); P <0.0001) but does not affect the mean lifespan of animals carrying the m540 or rh50 alleles of daf-9 ( d ); P =0.02 and P= 0.126, respectively). ( e ) eat-2(ad1116);daf-9(rh50) double mutants and daf-9(rh50) single mutants exhibit similar mean lifespans ( P =0.05). ( f ) Addition of 100 nM Δ 7 -DA does not affect the lifespan of wild-type animals under AL or BD conditions but restores the lifespan extension of daf-9(rh50) mutants ( P <0.0001). P values for survival analysis were calculated using the log-rank (Mantel–Cox) test. P values for QRT–PCR data were calculated using the two-tailed Student’s t -test; Error bars represent s.d. Lifespan values indicate mean±95% CI. Full size image DR-dependent steroid signalling extends lifespan To determine whether DAs were essential for DR-mediated longevity, we examined the lifespan of wild-type and daf-9 mutant animals [7] using two distinct DR paradigms. Complete removal of bacteria prolonged the lifespan of wild-type animals (ref. 8 , Fig. 1c and Supplementary Table 1 ) but not of two mutants carrying different loss-of-function alleles of daf-9 ( rh50 and m540 , Fig. 1d and Supplementary Table 1 ). Importantly, the two daf-9 mutants exhibited normal pharyngeal pumping rates ( Supplementary Fig. 3 ) and attraction to food (data not shown), excluding the possibility that they were constitutively nutrient deprived [9] . For the second DR paradigm, we introgressed the daf-9(rh50) allele into eat-2(ad1116) mutant worms. eat-2(ad1116) mutants are impaired in pharyngeal pumping and ingest bacteria at a slower pace, thus providing a bona fide genetic surrogate for DR [10] . eat-2(ad1116);daf-9(rh50) double mutants exhibited a lifespan comparable to that of daf-9(rh50) mutants and shorter than that of eat-2(ad1116 ) mutants ( Fig. 1e and Supplementary Table 1 ), demonstrating that the requirement for daf-9 activity was not restricted to the bacterial deprivation DR paradigm. We excluded the possibility that daf-9(rh50) mutants were constitutively unable to undergo lifespan extension by treating them with double-stranded RNA against the insulin receptor daf-2 , an intervention that increases longevity independently of DR. Under these conditions, we saw no difference in the lifespans of daf-2 RNA interference (RNAi) wild-type animals and similarly treated daf-9(rh50) mutants ( Supplementary Fig. 4 and Supplementary Table 1 ). To confirm that the requirement for daf-9 was linked to the production of DAs, we examined the lifespans of daf-9(rh50) mutants after supplementation with Δ 7 -DA. Notably, this treatment rescued the DR longevity response of daf-9(rh50) mutant animals to that seen with wild-type animals ( Fig. 1f and Supplementary Table 1 ). This suggests that, although daf-9(rh50) is considered to be a weak allele of daf-9 , Δ 7 -DA is sufficiently limiting in these animals to prevent their response to DR. Thus, DAs are produced by C. elegans in response to food deprivation and are required for lifespan extension through DR. To determine whether other steroidogenic genes might be involved in DR-mediated lifespan extension, we examined the role of several genes situated upstream of daf-9 , including daf-36 , emb-8 , dhs-16 and hsd-1 (refs 11 , 12 ). We found that these genes were dispensable for DR-induced lifespan extension ( Supplementary Fig. 5 and Supplementary Table 1 ), consistent with the notion proposed by others that DAs can be produced through an as yet uncharacterized alternative pathway [12] , [13] . Finally, we asked whether overproduction of DAs could enhance the response to bacterial deprivation. However, we found no significant differences in the lifespans of nutrient-deprived Δ 7 -DA–treated wild-type animals and animals overexpressing daf-9 compared with untreated wild-type animals ( Fig. 1f , Supplementary Fig. 6 and Supplementary Table 1 ). These data suggest that DAs are required, but not sufficient, for diet-mediated longevity enhancement. NHR-8 but not DAF-12 is required for lifespan extension In the canonical steroid-signalling pathway, DAs produced by DAF-9 binds to the nuclear hormone receptor, DAF-12. However, we found that daf-12(rh61rh411) null mutants also lived longer on DR ( Fig. 2a and Supplementary Table 1 ), suggesting that DAs can mediate this response in the absence of DAF-12. The C. elegans genome contains a second, closely related nuclear hormone receptor, NHR-8/NHR, which was recently shown to be involved in sterol homeostasis [14] and might therefore affect lifespan extension on DR. Under cholesterol-deficient conditions, animals carrying an nhr-8/ NHR null mutation exhibit phenotypes reminiscent of DA deficiency; for example, facilitated dauer formation, gonadal migration defects and a short lifespan [14] . Consistent with the notion that NHR-8 controls sterol production and homeostasis, these phenotypes could be rescued by supplementation with any sterol in the steroid-signalling pathway. We therefore asked whether NHR-8/NHR might also be involved in lifespan extension induced by DR. To bypass potentially confounding effects of nhr-8/ NHR deficiency on development, we used the weak ok186 allele of nhr-8/ NHR (deletion within the ligand-binding domain) and provided the animals with a standard concentration of cholesterol (5 μg·ml −1 ). Under these conditions, the nhr-8(ok186) mutants displayed no developmental defect or delay, but they did not undergo DR-induced lifespan extension ( Fig. 2b and Supplementary Table 1 ). Moreover, RNAi against nhr-8/ NHR from the first day of adulthood abrogated the long lifespan of eat-2(ad1116 ) mutants ( Supplementary Fig. 7 and Supplementary Table 1 ), confirming that nhr-8/ NHR is required to respond to both DR paradigms. Surprisingly, the addition of Δ 7 -DA had no effect on the lifespan of either fed or starved nhr-8(ok186) mutants ( Fig. 2c and Supplementary Table 1 ), suggesting that, in this context, Δ 7 -DA acts upstream of NHR-8. To further investigate the interaction between NHR-8 and Δ 7 -DA, we combined the daf-12(rh61rh411) and nhr-8(ok186) alleles with the daf-9(rh50) allele. We found that daf-12(rh61rh411);daf-9(rh50) double mutants could respond to DR only when Δ 7 -DA was provided ( Fig. 2d and Supplementary Table 1 ), whereas daf-9(rh50);nhr-8(ok186) double mutants failed to respond, even in the presence of Δ 7 -DA ( Fig. 2e and Supplementary Table 1 ). Similarly, DR did not induce lifespan extension in daf-12(rh61rh411);nhr-8(ok186) double mutants whether or not Δ 7 -DA was added ( Supplementary Fig. 8 and Supplementary Table 1 ). To ensure that our results did not simply reflect a general inability of nhr-8(ok186) mutants to undergo lifespan extension, we examined their response to daf-2 RNAi. This treatment extended the lifespan of control animals and nhr-8(ok186) mutants to a similar extent ( Supplementary Fig. 9 and Supplementary Table 1 ). Taken together, our results suggest that NHR-8, but not DAF-12, acts downstream of Δ 7 -DA to regulate DR. Thus, NHR-8/NHR has at least two independent functions in C. elegans . One is the regulation of larval development, which is observed in nhr-8/ NHR-null mutants under cholesterol-deficient conditions and is rescued by any sterol, including Δ 7 -DA [15] . The second is in DR-induced longevity, which is observed in animals carrying weak nhr-8/ NHR alleles and is not rescued by Δ 7 -DA ( Fig. 2c–e , Supplementary Fig. 8 and Supplementary Table 1 ). 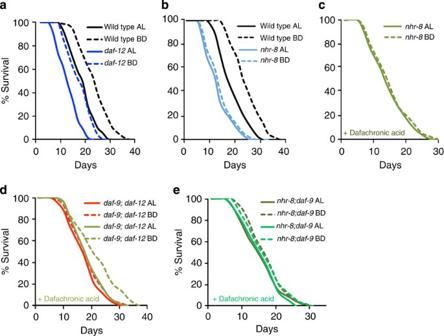Figure 2: NHR-8/NHR but not DAF-12 is required for dietary restriction-mediated lifespan extension. (a) Bacterial deprivation extends the lifespan ofdaf-12(rh61rh411)mutant animals by 27% (P<0.0001), similar to the effect on wild-type animals. (b) Bacterial deprivation does not affect the mean lifespan ofnhr-8(ok186)mutant animals (P=0.223). (c,d) Addition of 100 nM Δ7-DA does not restore DR-induced lifespan extension ofnhr-8(ok186)mutant animals (c); mean lifespans: BD, 17±1 days and AL, 17±1 days,P=0.642) but does that ofdaf-9(rh50);daf-12(rh61rh411)double mutants (d) BD, 19±1 days and AL, 22±1 days,P<0.0001). (e) In contrast, 100 nM Δ7-DA has no effect on the lifespan ofdaf-9(rh50);nhr-8(ok186)mutants (AL, 17±1 days and BD, 18±1 days,P=0.285).Pvalues were calculated using the log-rank (Mantel–Cox) test. Lifespan values represents mean±95% CI. Figure 2: NHR-8/NHR but not DAF-12 is required for dietary restriction-mediated lifespan extension. ( a ) Bacterial deprivation extends the lifespan of daf-12(rh61rh411) mutant animals by 27% ( P <0.0001), similar to the effect on wild-type animals. ( b ) Bacterial deprivation does not affect the mean lifespan of nhr-8(ok186) mutant animals ( P =0.223). ( c , d ) Addition of 100 nM Δ 7 -DA does not restore DR-induced lifespan extension of nhr-8(ok186) mutant animals ( c ); mean lifespans: BD, 17±1 days and AL, 17±1 days, P =0.642) but does that of daf-9(rh50);daf-12(rh61rh411) double mutants ( d ) BD, 19±1 days and AL, 22±1 days, P <0.0001). ( e ) In contrast, 100 nM Δ 7 -DA has no effect on the lifespan of daf-9(rh50);nhr-8(ok186) mutants (AL, 17±1 days and BD, 18±1 days, P =0.285). P values were calculated using the log-rank (Mantel–Cox) test. Lifespan values represents mean±95% CI. Full size image Our data show that lifespan extension induced by nutrient deprivation requires both NHR-8/NHR and Δ 7 -DA and that NHR-8 acts downstream of Δ 7 -DA; however, it is not yet clear whether Δ 7 -DA activates NHR-8 directly or indirectly. Indeed, in HEK293 cells, neither Δ 4 -DA nor Δ 7 -DA is able to transactivate NHR-8/NHR [7] . Three scenarios are compatible with our observations. First, NHR-8 could be activated by another form of DA. This is supported by a recent report that a variety of DAs can bind with different affinities and activate DAF-12 in vivo [13] . Second, NHR-8 activation could require binding with co-activators that are present in the worm, but not in HEK293 cells. Finally, DA could activate NHR-8 through one or more unidentified factors. Further investigation will be necessary to determine how Δ 7 -DA activates NHR-8/NHR in C. elegans . TOR signalling is controlled by steroid signalling To understand why animals deficient in daf-9(rh50) and/or nhr-8(ok186) /NHR failed to respond to DR, we examined several genes previously shown or suggested to be DR mediators [15] . The forkhead transcription factor PHA-4/FOXA is required for DR-mediated lifespan extension, and pha-4 messenger RNA (mRNA) levels are increased in eat-2(ad1116) -mutant animals [16] . However, pha-4 mRNA was induced to similar levels in daf-9(rh50) mutant and wild-type animals on food deprivation ( Supplementary Fig. 10 ). Similarly, induction of the b isoform of the zinc-finger transcription factor SKN-1/NRF2 in ASI neurons is necessary for diet-mediated longevity [17] . Here too, we found that lowering daf-9 mRNA levels (via RNAi) had no effect on GFP induction in nutrient-deprived skn-1b ::GFP animals ( Supplementary Fig. 11 ). The energy sensor aak-2 /AMPK is not only required for lifespan extension in response to DR [18] but overexpression results in significant lifespan extension [19] . We found that daf-9 RNAi had no effect on the AMP/ATP ratio in either fed or food-deprived wild-type and aak-2 /AMPK-overexpressing animals ( Supplementary Fig. 12b ). In addition, daf-9 RNAi effectively repressed the lifespan of eat-2 -mutant animals ( Supplementary Fig. 7a and Supplementary Table 1 ) but had no effect on that of aak-2 /AMPK-overexpressing animals ( Supplementary Fig. 12a and Supplementary Table 1 ). Collectively, these results strongly suggest that the responses of pha-4 , skn-1b and aak-2 mutants to DR are not affected by steroid signalling. Since these genes were shown to mediate DR-mediated lifespan extension, our data raise the possibility that lifespan extension of wild-type animals through DR can also occur independent of steroid signalling. We therefore searched for genes linked to lifespan regulation through steroid signalling. Downregulation of the target of rapamycin (tor) gene, let-363 , through genetic ablation [20] , [21] , [22] , RNAi [21] , or chemical inactivation [23] , has been shown to decrease TOR signalling and extend the lifespan of yeast [20] , flies [22] , worms [21] and mice [23] , [24] . Because TOR is a nutrient-sensing kinase, we considered that it may play a role in promoting the longevity response to DR. Indeed, nutrient deprivation markedly decreased let-363 /mTOR mRNA levels in wild-type animals ( Fig. 3a ). However, DR did not affect let-363 /mTOR mRNA levels in either daf-9(rh50) mutants or nhr-8(ok186) mutants and had an intermediate effect in daf-12(rh61rh411) mutants ( Fig. 3a ). Consistent with the results of our lifespan analysis, addition of Δ 7 -DA did not further reduce let-363 /mTOR mRNA levels in nutrient-deprived wild-type animals ( Fig. 3b ). Δ 7 -DA did, however, reduce let-363 /mTOR mRNA levels in nutrient-deprived daf-9(rh50) and daf-12(rh61rh411) mutants to the levels observed in wild-type animals ( Fig. 3b ). In contrast, Δ 7 -DA had no effect on let-363 /mTOR levels in nhr-8(ok186) mutants, suggesting that Δ 7 -DA may regulate let-363 /mTOR mRNA levels through NHR-8/NHR ( Fig. 3b ). On Δ 7 -DA supplementation, daf-9(rh50);daf-12(rh61rh411) double mutants subjected to DR exhibited low let-363 /mTOR levels ( Supplementary Fig. 13 ) and an extended lifespan ( Fig. 2d ), whereas daf-9(rh50);nhr-8(ok186) double mutants harboured high let-363 /mTOR mRNA levels ( Supplementary Fig. 13 ) and remained unable to respond to DR ( Fig. 2e ). These data raise the possibility that the high let-363 /TOR mRNA levels in daf-9 and nhr-8 mutants prevent their response to DR. To test this hypothesis, we determined whether reducing let-363 /mTOR expression would extend the lifespan of eat-2(ad1116);daf-9(rh50) double mutants, which are normally unresponsive to DR. Indeed, let-363 RNAi increased the mean lifespan of the double mutants to that of the eat-2 single mutants, suggesting that high let-363 /mTOR levels prevented DR-mediated lifespan extension in these animals ( Fig. 3c and Supplementary Table 1 ). 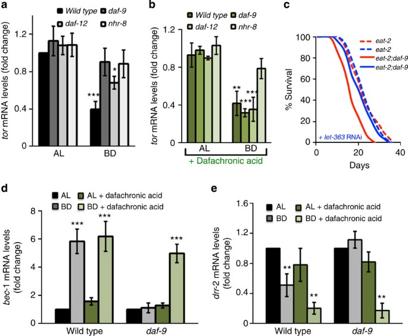Figure 3:let-363/mTORresponds to nutrient availability in a steroid hormone-dependent manner. (a)let-363mRNA levels are reduced upon nutrient deprivation in wild-type worms (60%, ΔΔCt=1.33 normalized to AL;P<0.001,n=6 independent biological samples) but not indaf-9(rh50)ornhr-8(ok186)-mutant animals (P=0.362 andP=0.068, respectively,n=6 independent biological samples for each). Nutrient deprivation has an intermediate effect onlet-363/mTOR mRNA levels indaf-12(rh61rh411)mutants (37.25%; ΔΔCt=0.55 normalized to AL,P<0.01,n=6 independent biological samples). (b) Supplementation with 100 nM Δ7-DA decreaseslet-363mRNA levels by 50%, 66%, and 54% in wild-type,daf-9(rh50)mutant, anddaf-12(rh61rh411)mutant animals, respectively, but had no effect onnhr-8(ok186)mutants (P=0.054,n=6 independent biological samples). (c) RNAi-mediated downregulation oflet-363extends the lifespan ofeat-2(ad1116);daf-9(rh50)double mutants (29%,P<0.001) to the levels ofeat-2(ad1116)single mutants but fails to extend the lifespan ofeat-2(ad1116)single mutants. Pvalues for mRNA quantification and lifespan analyses were calculated using the two-tailed Student’st-test and log-rank (Mantel–Cox) test, respectively. (d) Nutrient deprivation induces TOR signalling, as shown by increased transcription of the autophagy genebec-1, in wild-type animals (600%, ΔΔCt=−2.54 normalized to AL,P<0.001,n=5 independent biological samples) but not indaf-9(rh50)mutants (6%,P=0.474,n=6 independent biological samples). Supplementation with 100 nM Δ7-DA restores wild type-like induction ofbec-1transcription indaf-9(rh50)mutants (500%, ΔΔCt=−2.31 normalized to AL,P<0.001,n=6 independent biological samples) (e) Nutrient deprivation reduces expression of the elongation factordrr-2in wild-type animals (−50%, ΔΔCt=0.97 normalized to AL,P<0.01,n=5 independent biological samples) but not indaf-9(rh50)mutants (P=0.386,n=6 independent biological samples). Addition of 100 nM Δ7-DA restores wild type-likedrr-2transcript levels indaf-9(rh50)mutants (−80%, ΔΔCt=2.52 normalized to AL,P<0.001,n=6 independent biological samples).Pvalues were calculated using the two-tailed Student’st-test. Error bars represent s.d. Figure 3: let-363/mTOR responds to nutrient availability in a steroid hormone-dependent manner. ( a ) let-363 mRNA levels are reduced upon nutrient deprivation in wild-type worms (60%, ΔΔCt=1.33 normalized to AL; P <0.001, n =6 independent biological samples) but not in daf-9(rh50) or nhr-8(ok186) -mutant animals ( P =0.362 and P =0.068, respectively, n =6 independent biological samples for each). Nutrient deprivation has an intermediate effect on let-363 /mTOR mRNA levels in daf-12(rh61rh411) mutants (37.25%; ΔΔCt=0.55 normalized to AL, P <0.01, n =6 independent biological samples). ( b ) Supplementation with 100 nM Δ 7 -DA decreases let-363 mRNA levels by 50%, 66%, and 54% in wild-type, daf-9(rh50) mutant, and daf-12(rh61rh411) mutant animals, respectively, but had no effect on nhr-8(ok186) mutants ( P =0.054, n =6 independent biological samples). ( c ) RNAi-mediated downregulation of let-363 extends the lifespan of eat-2(ad1116);daf-9(rh50) double mutants (29%, P <0.001) to the levels of eat-2(ad1116) single mutants but fails to extend the lifespan of eat-2(ad1116) single mutants . P values for mRNA quantification and lifespan analyses were calculated using the two-tailed Student’s t -test and log-rank (Mantel–Cox) test, respectively. ( d ) Nutrient deprivation induces TOR signalling, as shown by increased transcription of the autophagy gene bec-1 , in wild-type animals (600%, ΔΔCt=−2.54 normalized to AL, P <0.001, n =5 independent biological samples) but not in daf-9(rh50) mutants (6%, P =0.474, n =6 independent biological samples). Supplementation with 100 nM Δ 7 -DA restores wild type-like induction of bec-1 transcription in daf-9(rh50) mutants (500%, ΔΔCt=−2.31 normalized to AL, P <0.001, n =6 independent biological samples) ( e ) Nutrient deprivation reduces expression of the elongation factor drr-2 in wild-type animals (−50%, ΔΔCt=0.97 normalized to AL, P <0.01, n =5 independent biological samples) but not in daf-9(rh50) mutants ( P =0.386, n =6 independent biological samples). Addition of 100 nM Δ 7 -DA restores wild type-like drr-2 transcript levels in daf-9(rh50) mutants (−80%, ΔΔCt=2.52 normalized to AL, P <0.001, n =6 independent biological samples). P values were calculated using the two-tailed Student’s t -test. Error bars represent s.d. Full size image Collectively, our data show that the transcription of let-363 /mTOR is regulated by both nutrients and Δ 7 -DA (or a derived metabolite) and suggest that integration of the nutritional and steroidal signals occurs via NHR-8/NHR. Whether NHR-8/NHR controls let-363 /mTOR expression directly or indirectly remains to be determined. We verified that altered let-363 /TOR expression was sufficient to perturb TOR signalling in daf-9(rh50) mutants. For this, we measured expression of the autophagy genes, bec-1, atg-18 , which are induced by DR, and of the translation gene, drr-2 , which is reduced by DR in a TOR signalling-dependent manner. We found that bec-1 and atg-18 mRNA levels were enhanced, whereas drr-2 mRNA was reduced, by nutrient deprivation in wild-type animals but not in daf-9(rh50) mutants, consistent with aberrant TOR signalling in these animals ( Fig. 3d,e and Supplementary Fig. 14 ). Convincingly, addition of exogenous Δ 7 -DA was sufficient to restore wild type-like levels of bec-1 and drr-2 mRNA in daf-9(rh50) mutants ( Fig. 3d,e ). We also analysed animals expressing a GFP-tagged version of the LC3 ortholog, LGG-1 and confirmed that daf-9 RNAi impairs autophagosome formation in these animals under DR conditions ( Supplementary Fig. 14 ). Thus, Δ 7 -DA (or a derived metabolite) acts upstream of the nuclear receptor NHR-8/NHR, but not DAF-12, to regulate let-363 /mTOR expression and downstream processes. TOR is therefore capable of regulating longevity by integrating both nutrient-derived and steroidal signals in C. elegans at the transcriptional level. Germline plasticity is linked to lifespan extension TOR signalling was recently shown to control the proliferation of germ cells in the proliferative zone of the gonad and their entry into meiosis in response to nutrient availability [25] . We therefore tested the possibility that steroid signalling through the DAF-9/Δ 7 -DA/NHR-8 pathway may affect the response of the germline to DR. Indeed, we observed that nutrient deprivation significantly decreased the number of nuclei in the germline of wild-type animals but had no effect in either daf-9(rh50) or nhr-8(ok186) mutants ( Fig. 4a,b ). Notably, addition of Δ 7 -DA restored the number of nuclei to wild-type levels in daf-9(rh50) but not in nhr-8(ok186) mutants ( Fig. 4a,b ). This is consistent with the notion that low TOR levels are associated with low germ cell count [25] . To test the possibility that steroid signalling-dependent germline plasticity is linked to the lifespan extension conferred by DR, we combined the daf-9(rh50) and the nhr-8(ok186) alleles with the glp-1(e2141ts) and the daf-7(e1372) alleles, which alters germline stem cell proliferation through distinct pathways [26] . The glp-1(e2141ts) allele completely arrests germline stem cell proliferation at 25 °C but has only a partial effect at 20 °C. At this temperature, germline signalling is not active and glp-1(e2141ts) mutant animals display a wild type-like lifespan under both BD and ad libitum feeding conditions ( Fig. 5a and Supplementary Table 1 ). The C. elegans transforming growth factor DAF-7 also regulates germline plasticity. Downregulation of the TGF-β pathway also reduces the number of germ cells in the proliferative zone by promoting their differentiation, but this occurs in a glp-1 -independent manner [26] . We observed that daf-7(e1372);nhr-8(ok186) , glp-1(e2141ts);daf-9(rh50) and glp-1(e2141ts);nhr-8(ok186) double mutants raised at 20 °C did indeed have fewer nuclei in the distal part of the germline, and starvation further reduced this number ( Fig. 4c,d ). Interestingly, DR enhanced the lifespans of these animals normally ( Fig. 5b–d and Supplementary Table 1 ). 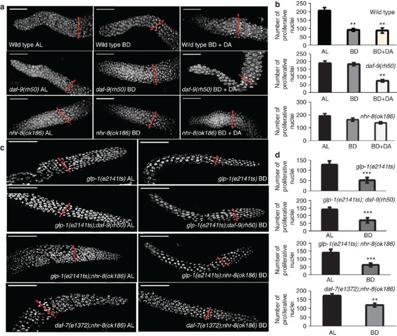Figure 4: During nutrient deprivation, steroid signalling controls germ cells number. (a) Imaging of the proliferative zone of the germline of wild-type,daf-9(rh50), andnhr-8(ok186)mutants fedad libitumor subjected to bacterial deprivation in the presence or absence of DA. Nuclei were stained with 4′,6-diamidino-2-phenylindole (DAPI). (b) Quantification of germ cells in the animals shown ina, indicating the lack of effect of DR on germ cell numbers indaf-9(rh50)andnhr-8(ok186)mutants (AL,n=11, 13, and 9, respectively for wild-type,daf-9(rh50), andnhr-8(ok186)mutants; BD,n=10, 12 and 10, respectively for wild-type,daf-9(rh50)andnhr-8(ok186)mutants). Addition of Δ7-DA reduced germ cells indaf-9(rh50), but notnhr-8(ok186)mutants (n=9, 11 and 9, respectively for wild-type,daf-9(rh50)andnhr-8(ok186)mutants). (c) Proliferative zone of the germline ofglp-1(e2141ts),glp-1(e2141ts);daf-9(rh50)andglp-1(e2141ts);nhr-8(ok186)mutants labelled with DAPI were imaged either fedad libitumor subjected to bacterial deprivation at 20 °C. (d) The quantification of the number of cells present in these animals show that in all strain analysed, germ cells number is decreased in response to nutrient deprivation.glp-1(e2141ts), glp-1(e2141ts);daf-9(rh50),glp-1(e2141ts);nhr-8(ok186)anddaf-7(e1372);nhr-8(ok186)mutants (AL, 128±17 proliferative nuclei and BD, 52±13 proliferative nuclei,P<0.0001 forglp-1(e2141ts), n=13 and 11 for AL and BD conditions, respectively; AL, 142±13 proliferative nuclei and BD, 70±17 proliferative nuclei,P<0.0001 forglp-1(e2141ts);daf-9(rh50), n=9 and 12 for AL and BD conditions, respectively; AL, 140±21 proliferative nuclei and BD, 62±10 proliferative nuclei,P<0.0001 forglp-1(e2141ts);nhr-8(ok186), n=11 and 9 for AL and BD conditions, respectively and AL, 172±12 proliferative nuclei and BD, 119±11 proliferative nuclei,P<0.01 fordaf-7(e1372);nhr-8(ok186)),n=10 and 8 for AL and BD conditions, respectively. Pvalues were calculated using the two-tailed Student’st-test. Scale bar, 40 μm. Error bars represent s.e.m. Figure 4: During nutrient deprivation, steroid signalling controls germ cells number. ( a ) Imaging of the proliferative zone of the germline of wild-type, daf-9(rh50) , and nhr-8(ok186) mutants fed ad libitum or subjected to bacterial deprivation in the presence or absence of DA. Nuclei were stained with 4′,6-diamidino-2-phenylindole (DAPI). ( b ) Quantification of germ cells in the animals shown in a , indicating the lack of effect of DR on germ cell numbers in daf-9(rh50) and nhr-8(ok186) mutants (AL, n =11, 13, and 9, respectively for wild-type, daf-9(rh50) , and nhr-8(ok186) mutants; BD, n =10, 12 and 10, respectively for wild-type, daf-9(rh50) and nhr-8(ok186) mutants). Addition of Δ 7 -DA reduced germ cells in daf-9(rh50) , but not nhr-8(ok186) mutants ( n =9, 11 and 9, respectively for wild-type, daf-9(rh50) and nhr-8(ok186) mutants). ( c ) Proliferative zone of the germline of glp-1(e2141ts) , glp-1(e2141ts);daf-9(rh50) and glp-1(e2141ts);nhr-8(ok186) mutants labelled with DAPI were imaged either fed ad libitum or subjected to bacterial deprivation at 20 °C. ( d ) The quantification of the number of cells present in these animals show that in all strain analysed, germ cells number is decreased in response to nutrient deprivation. glp-1(e2141ts), glp-1(e2141ts);daf-9(rh50) , glp-1(e2141ts);nhr-8(ok186) and daf-7(e1372);nhr-8(ok186) mutants (AL, 128±17 proliferative nuclei and BD, 52±13 proliferative nuclei, P <0.0001 for glp-1(e2141ts), n =13 and 11 for AL and BD conditions, respectively; AL, 142±13 proliferative nuclei and BD, 70±17 proliferative nuclei, P <0.0001 for glp-1(e2141ts);daf-9(rh50), n =9 and 12 for AL and BD conditions, respectively; AL, 140±21 proliferative nuclei and BD, 62±10 proliferative nuclei, P <0.0001 for glp-1(e2141ts);nhr-8(ok186), n =11 and 9 for AL and BD conditions, respectively and AL, 172±12 proliferative nuclei and BD, 119±11 proliferative nuclei, P <0.01 for daf-7(e1372);nhr-8(ok186) ), n =10 and 8 for AL and BD conditions, respectively . P values were calculated using the two-tailed Student’s t -test. Scale bar, 40 μm. Error bars represent s.e.m. 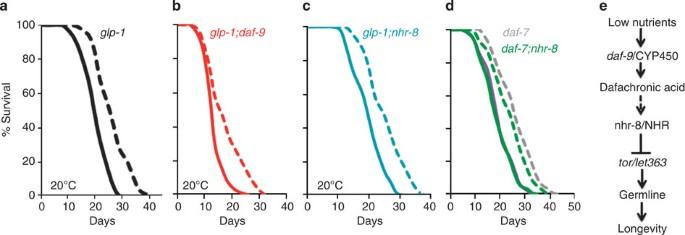Figure 5: Low germ cell count restores diet-induced lifespan extension indaf-9andnhr-8mutants. (a)glp-1(e2141ts)-mutant animals at 20 °C exhibit wild type-like mean lifespans underad libitumfeeding or BD conditions (mean lifespan: AL, 21±0.7 days and BD, 27±1 days,P<0001). (b–d) Restoration of DR-induced lifespan extension by genetically mimicking the effects of DR on germline plasticity with theglp-1(e2141ts)allele at 20 °C in combination with either the (b)daf-9(rh50)or (c) thenhr-8(ok186)alleles: (b)glp-1(e2141ts);daf-9(rh50)(mean lifespan: AL, 14±1 days and BD, 18±1.5 days,P<0001) and (c)glp-1(e2141ts);nhr-8(ok186)mutants (AL, 20±1 days and BD, 26±1 days,P<0.0001). (d) Similar results are obtained using thedaf-7(e1372)allele:daf-7(e1372);nhr-8(ok186)mutants (AL, 19±1 days and BD, 24±1 days,P<0.0001). For all lifespan curves, solid and dashed lines representad libitumand BD feeding conditions, respectively. (e) We propose a model in which nutrient scarcity induces DAF-9-mediated production of DA. In turn, DA activates NHR-8/NHR and TOR signalling, culminating in lifespan extension through the germline. The precise nature of the NHR-8/NHR ligand(s) and interactor(s) remains to be determined.Pvalues were calculated using the log-rank (Mantel–Cox) test for lifespan. Lifespan values indicate mean±95% CI. Full size image Figure 5: Low germ cell count restores diet-induced lifespan extension in daf-9 and nhr-8 mutants. ( a ) glp-1(e2141ts) -mutant animals at 20 °C exhibit wild type-like mean lifespans under ad libitum feeding or BD conditions (mean lifespan: AL, 21±0.7 days and BD, 27±1 days, P <0001). ( b – d ) Restoration of DR-induced lifespan extension by genetically mimicking the effects of DR on germline plasticity with the glp-1(e2141ts) allele at 20 °C in combination with either the ( b ) daf-9(rh50) or ( c ) the nhr-8(ok186) alleles: ( b ) glp-1(e2141ts);daf-9(rh50) (mean lifespan: AL, 14±1 days and BD, 18±1.5 days, P <0001) and ( c ) glp-1(e2141ts);nhr-8(ok186) mutants (AL, 20±1 days and BD, 26±1 days, P <0.0001). ( d ) Similar results are obtained using the daf-7(e1372) allele: daf-7(e1372);nhr-8(ok186) mutants (AL, 19±1 days and BD, 24±1 days, P <0.0001). For all lifespan curves, solid and dashed lines represent ad libitum and BD feeding conditions, respectively. ( e ) We propose a model in which nutrient scarcity induces DAF-9-mediated production of DA. In turn, DA activates NHR-8/NHR and TOR signalling, culminating in lifespan extension through the germline. The precise nature of the NHR-8/NHR ligand(s) and interactor(s) remains to be determined. P values were calculated using the log-rank (Mantel–Cox) test for lifespan. Lifespan values indicate mean±95% CI. Full size image Taken together, the results presented here demonstrate that steroid signalling is activated by nutrient scarcity and is required for DR effects on lifespan extension through TOR signalling. In the absence of proper steroid signalling, let-363 /mTOR levels remain high during starvation ( Fig. 3a ) and the number of germ cells within the proliferative zone of the germline is no longer affected by nutrient availability ( Fig. 4 ). Interestingly, genetic reduction of germ cells alleviates the requirement for steroid signalling for DR-mediated lifespan extension. We speculate that genetically lowering the germ cell count mimics the response of the germline to DR and induces a signal that is usually emitted when nutrients are scarce and the germline becomes less active. In wild-type animals, this would normally be achieved through the DAF-9/Δ 7 -DA/NHR-8 pathway. However, further work will be necessary to confirm the identity of this signal. It is important to note that bacterial deprivation also extends the lifespan of sterile or post-reproductive animals [27] , [28] . In these animals, the putative signal for low germline activity might be constitutively produced, resulting in activated steroid signalling. Alternative mechanisms may also contribute to DR-induced longevity when reproduction is fully extinguished. Interestingly, recent studies have shown that the mammalian lifespan-promoting hormone FGF21 (ref. 29 ) also controls female reproduction [30] and that its expression is regulated by the nuclear hormone receptors farnesoid X receptor and liver X receptor, both of which are NHR homologues, and is induced by bile acids similar to Δ 7 -DA [31] , [32] . Our findings therefore establish the molecular basis for the interplay between nutrition and reproduction in regulating lifespan. Strains Strains used in this study include N2, daf-9(rh50), daf-9(m540), daf-12(rh61rh411), daf-7(e1372), nhr-8(ok186), daf-9(e1406);mgEx662[daf-9p::daf-9 genomic::GFP], eat-2(ad1116) , HGA8015 [eat-2(ad1116);daf-9(rh50)] , glp-1(e2141ts);daf-9(rh50) , HGA8016 [nhr-8(ok186);daf-9(rh50)] , HGA8017 [daf-12(rh61rh411);nhr-8(ok186)] , HGA8018 [daf-7(e1372);nhr-8(ok186)] , HGA8019 [glp-1(e2141ts);nhr-8(ok186)] and daf-12(rh61rh411);daf-9(rh50) . Lifespan analyses For lifespan analyses, synchronized L1 larvae were raised at 20 °C until they reached the late L4 larval stage or early day 1 of adulthood. Worms were then transferred to NGM plates containing 5-fluorouracil (to prevent development of progeny) with or without bacteria. Statistical analysis of lifespan data was performed with XLSTAT software (Addinsoft). RNAi experiments were performed by substituting control bacteria with bacteria carrying a vector carrying a RNAi clone [33] . Real-time QPCR Real-time quantitative PCR experiments were performed using a standard protocol with FastStart SYBR Green Master Mix and the StepOne Plus system (Applied Biosystems). Microscopy Images of SKN-1::GFP worms were acquired with a Nikon fluorescent microscope at × 400 magnification, and signals were quantified using ImageJ software (NIH). DA treatment For DA treatment, Δ 7 -DA (Adipogen) was dissolved in ethanol and added to NGM plates at a final concentration of 100 nM. DA measurement DA was measured by reversed-phase UPLC followed by mass spectrometry in negative ionization mode. Approximately 20,000 worms (~5 mg protein) were washed from the cultivation plates with cold phosphate-buffered saline. After addition of 2 ml methanol, worms were lysed by sonication in a water bath at 4 °C for 15 min. Samples were centrifuged at 14,000 r.p.m. and 4 °C for 10 min, the supernatant was transferred to a fresh tube, and the solvent was evaporated using a SpeedVac concentrator. The residue was dissolved in 100 μl methanol and the sample was separated on a Phenomenex Kinetex C18 column (50 mm × 2.1 mm, 1.3 μm particle size) with an acetonitrile gradient. Separation was carried out on a Waters Acquity UPLC (Waters) coupled to a Bruker maXis UHR-ToF-MS (Bruker Daltonics). The system was calibrated using Low Concentration Tuning Mix (Agilent). Samples were quantified by external calibration with a Δ 7 -DA standard (Biomol) in the range 0 to 2.5 μg/ml DA. R 2 for calibration was >0.9. AMP/ATP measurement Worms were washed twice with S-buffer to remove bacteria and waste products, transferred to a 15 ml tube, and resuspended in 4 ml of S-buffer. Remaining bacteria were removed by addition of 8 ml of 60% sucrose followed by thorough shaking and centrifugation for 1 min at 3,000 r.p.m. The nematodes were then transferred to a fresh 15 ml tube and washed twice more with S-buffer. The supernatant was removed and the worm pellet (~100 μl) was mixed with glass beads (0.2 g) and homogenized using a mechanical bead beater. The homogenate was centrifuged (8–10 min, 4 °C, 14,000 r.p.m.) and the supernatant was transferred to a fresh 1.5 ml tube. The ADP/ATP ratio in 10 μl aliquots of worm extract was measured with an EnzyLight ADP/ATP Ratio Assay kit (ELDT-100, BioAssay Systems), according to the manufacturer’s procedure. EnzyLight assay data were normalized to the total protein content of worm samples, as determined with the Bradford protein assay. The AMP/ATP ratio was approximated as the square of the ADP/ATP ratio [34] . Germ cell count The number of cells in the proliferative zone was assessed as described. Briefly, adult worms (day 2) were immobilized on a microscope slide using levamisole solution (0.2 mM in M9). Gonads were extruded by cutting the worms at the head near the pharyngeal bulb or at the anal region. Worms with extruded gonads were fixed in cold methanol for 5 min and washed by the addition of PBTw (1 × phosphate-buffered saline with 0.1% Tween 20) followed by centrifugation at 3,000 r.p.m. for 1 min. The supernatant was discarded and the worms were washed twice more. The worm pellet was then incubated with 4′,6-diamidino-2-phenylindole solution (100 ng ml −1 ) for 1 min, transferred onto a large 2% agarose pad and covered with a coverslip. Images were acquired using a confocal Leica TCS SP5 microscope with × 40 or × 63 zoom lenses (final zoom × 400 or × 630). To enumerate germ cells, the boundary between the mitotic and transition zones was marked as described by Crittenden et al . [35] Cells in the proliferative zone were counted at different focal planes through the width of the germline. Pumping rate Animals were raised at 20 °C until they reached late L4 larval stage or early day 1 of adulthood. Animals were then transferred to NGM plates with or without bacteria and pharyngeal pumping was evaluated on the second day of adulthood. Animals were left undisturbed for 1 h and pharyngeal pumping was counted for 20 s in at least 20 worms for each condition. Results are presented as the mean±s.d. and statistical significance was analysed using Student’s t -test. Quantitative PCR Synchronized L1 larvae were grown at 20 °C on HT115 Escherichia coli until they reached late L4 stage or early day 1 of adulthood. Animals were then transferred to NGM plates with or without bacteria. For RNAi experiments, animals were raised at 20 °C on HT115 E. coli bacteria and were transferred onto plates seeded with control bacteria or bacteria expressing double-stranded RNA against the gene of interest. On day 2 of adulthood, animals were collected and washed three times with M9 solution. Washed animals (~1,000 per point) were frozen at −80 °C for at least 24 h. RNA was extracted using TRIzol (Invitrogen) and RNeasy Mini Kits (Qiagen). The concentration and purity of RNA was determined using a NanoDrop spectrophotometer. cDNA was synthesized from samples of 1 μg of RNA using an iScript Advanced cDNA Synthesis Kit (Bio-Rad). QPCR was performed using the StepOne Plus system (Applied Biosystems) according to the manufacturer’s recommended protocol. Relative mRNA levels were normalized against the housekeeping genes cdc-42 , pmp-3 and ama-1 . Primers are listed in Supplementary Table 2 . Results are expressed as the mean±s.d. of triplicates. All QPCR experiments are repeated at least 2times. Statistical significance was determined using the two-tailed Student’s t -test. How to cite this article : Thondamal, M. et al . Steroid hormone signalling links reproduction to lifespan in dietary-restricted Caenorhabditis elegans . Nat. Commun. 5:4879 doi: 10.1038/ncomms5879 (2014).